A competitive and reversible deactivation approach to catalysis-based quantitative assays Catalysis-based signal amplification makes optical assays highly sensitive and widely useful in chemical and biochemical research. However, assays must be fine-tuned to avoid signal saturation, substrate depletion and nonlinear performance. Furthermore, once stopped, such assays cannot be restarted, limiting the dynamic range to two orders of magnitude with respect to analyte concentrations. In addition, abundant analytes are difficult to quantify under catalytic conditions due to rapid signal saturation. Herein, we report an approach in which a catalytic reaction competes with a concomitant inactivation of the catalyst or consumption of a reagent required for signal generation. As such, signal generation proceeds for a limited time, then autonomously and reversibly stalls. In two catalysis-based assays, we demonstrate restarting autonomously stalled reactions, enabling accurate measurement over five orders of magnitude, including analyte levels above substrate concentration. This indicates that the dynamic range of catalysis-based assays can be significantly broadened through competitive and reversible deactivation. Development of optical assays for facile quantification of trace analytes is an ever-expanding field. Target analytes range from trace metals [1] and biological signalling agents [2] , [3] to chemical weapons [4] . Tailored chemosensors interact specifically with an analyte to produce an optically decoded signal, which can manifest itself as a wavelength shift or intensity change in either absorbance or emission. These signals are measured by simple instrumentation, such as a plate reader, or visualized with the naked eye. Quantitative optical assays exploit either a catalytic or a non-catalytic reaction. Non-catalytic assays rely on a single turnover from the analyte for a chemical conversion or a reversible binding and have the benefit of time-independence; in other words, the signal does not change over time once the reaction or binding event is complete. A major drawback of these systems is the higher limits of quantification due to this limited turnover, rendering these non-catalytic assays undesirable for detection of trace analytes. A more sensitive approach for trace analytes uses catalysis-based assays, where the substrate continues to react over time, amplifying signals. The continuity of catalysis-based signal amplification presents some practical challenges to assay development. In metal catalysis-based assays, once the metal has entered into the catalytic cycle, the resulting fluorescence signal is dependent on the concentration of the analyte as well as the time elapsed, with the reaction continuing until the fluorogenic substrate is consumed. In enzyme and enzyme-linked immunosorbent assays [5] , the reaction continues until the substrate is consumed or a terminating reagent is added [6] . In either case, if an analyte is abundant, the assay substrate will be rapidly consumed, preventing accurate quantitation. In addition, if a reaction with a low concentration of analyte is allowed to continue unchecked, the signal can increase to the point where the detector becomes saturated, again preventing accurate quantification. Finally, when a catalysis-based assay is externally stopped, it cannot be restarted [6] and premature termination requires the assay to be repeated to obtain quantitative data. As such, a significant drawback associated with catalysis-based assays is the far narrower dynamic range (one to two orders of magnitude) compared with more labour-intensive methods, such as inductively coupled plasma mass spectrometry (ICP-MS), which has a detection range is up to five orders of magnitude. New methodologies that overcome these limitations to enable controlled activity of catalytic assays would be broadly useful in chemical and biochemical research. Herein, we present a new approach to catalysis-based assays in which a catalytic chromogenic reaction competes with the deactivation of the catalyst or depletion of an essential reagent. Under these conditions, a signal-producing reaction proceeds for a limited time, then autonomously stalls, but can be reactivated by reagent addition, generating a graph reminiscent of a staircase function in mathematics. This approach is exemplified by both a new colorimetric method for quantifying palladium (Pd) and a horseradish peroxidase assay system. In the analysis of Pd, multiple cycles of reaction stalling and restarting allow accurate measurement with a detection range of over five orders of magnitude. Moreover, analyte levels significantly above the substrate concentration can be quantified. Resorufin allyl ether as a chemodosimeter for palladium We previously reported a fluorescence method for quantifying Pd in pharmaceuticals based on the Pd-catalysed fluorogenic conversion of allyl Pittsburgh Green ether (APE) to Pittsburgh Green ( Fig. 1a ) [7] , [8] , [9] , [10] . Although this method showed excellent sensitivity and an ability to accurately quantify low-level Pd in real-world samples, we realized that a colorimetric version of the assay could allow even simpler, instrument-free access to low-level Pd measurements, a goal previously attempted by several other researchers with limited success [11] , [12] . 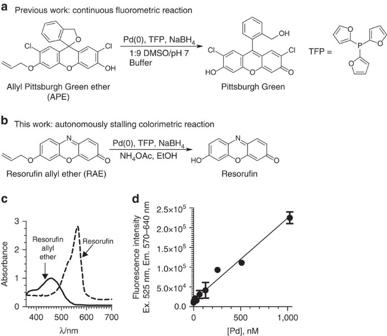Figure 1: Palladium chemodosimeters based on change in optical properties. (a) Structures of previously developed fluorogenic chemodosimeter APE and its conversion to Pittsburgh Green. (b) Chromogenic chemodosimeter RAE and its conversion to resorufin. (c) Absorption spectra of resorufin and RAE in 800 mM NH4OAc in EtOH. The data are normalized to 20 μM of each compound. (d) Correlation between Pd concentrations and fluorescence signal using RAE.r2=0.97,y=(208±7.38)x+(15,910±2,765). Conditions: 29 μM RAE, 0, 8, 16, 32, 64, 128, 256, 512, 1,024 nM Pd(II). 50 mM NaBH4, 200 μM TFP, 800 mM NH4OAc, EtOH, 24 °C, 60 min;n=3. Figure 1: Palladium chemodosimeters based on change in optical properties. ( a ) Structures of previously developed fluorogenic chemodosimeter APE and its conversion to Pittsburgh Green. ( b ) Chromogenic chemodosimeter RAE and its conversion to resorufin. ( c ) Absorption spectra of resorufin and RAE in 800 mM NH 4 OAc in EtOH. The data are normalized to 20 μM of each compound. ( d ) Correlation between Pd concentrations and fluorescence signal using RAE. r 2 =0.97, y =(208±7.38) x +(15,910±2,765). Conditions: 29 μM RAE, 0, 8, 16, 32, 64, 128, 256, 512, 1,024 nM Pd(II). 50 mM NaBH 4 , 200 μM TFP, 800 mM NH 4 OAc, EtOH, 24 °C, 60 min; n =3. Full size image Investigation of a number of candidate chromogenic substrates led to the preparation of yellow-coloured resorufin allyl ether (RAE) in one step in 85% yield from commercially available purple-coloured resorufin ( Fig. 1b,c , Supplementary Figs 13 and 14 ). Attempts at Pd-catalysed deallylation of RAE using the optimized conditions for APE (tris(2-furyl)phosphine (TFP)), NaBH 4 , dimethyl sulphoxide (DMSO)/1.23 M phosphate pH 7 buffer (1:9)) were unsuccessful. However, screening a variety of commercially available phosphines and additives ( Supplementary Table S1 and Supplementary Figs 1–3 ) led to the identification of suitable conditions for carrying out the transformation. Optimized conditions for the Pd-dependent deallylation of RAE used TFP, NH 4 OAc and NaBH 4 in an EtOH solvent. Further optimization of RAE as a substrate can be found in the Supplementary Methods and Supplementary Figs 2–4 . We found that RAE was selectively responsive to Pd over other metals tested (Ag, Au, Cd, Co, Cr, Fe, Hg, Mn, Ni. Pt, Rh, Ru, Zn, Sr, Ir, Cu; Supplementary Fig. 4a,b ) and could detect Pd without interference from these metals, with the exception of Hg, where a small level of interference was observed ( Supplementary Fig. 4c ). When selectivity was tested by absorbance, higher values were observed in the presence of Au, Ag, and Hg owing to turbidity of the solution, although fluorescence measurement revealed that these were merely false positives (that is, these metals did not convert RAE to resorufin; Supplementary Fig. 4a,b ). When exposed to Pd, the fluorescence signal increased linearly with respect to Pd concentration ( Fig. 1d ), indicating a first-order relationship suitable for convenient quantification. The Pd-catalysed deallylation of APE in phosphate buffer was more effective in the presence of NaBH 4 , which reduces Pd(II) and Pd(IV) to catalytically active Pd(0), but did not require this reducing agent as a critical component [9] . In contrast, Pd(II) species did not catalyse the deallylation of RAE in NH 4 OAc-containing EtOH without the reducing agent, with the amount of NaBH 4 dictating the duration of reaction ( Fig. 2a ). This novel NaBH 4 -dependence boded well with our aim at competitively and reversibly deactivating catalysis-based assays, as detailed below. Lower concentrations of NaBH 4 , ranging from 5–25 mM, led to stalling of the colour-forming reaction within 30 s, presumably because of rapid consumption of the reductant, NaBH 4 , combined with ongoing air-oxidation of catalytically active Pd(0) to higher valent, inactive Pd species. In contrast, NaBH 4 concentrations in excess of 50 mM allowed the reaction to continue for several minutes. Importantly, the addition of more NaBH 4 could restart a stalled deallylation reaction ( Fig. 2b ), affording a convenient way to trigger signal generation on demand. 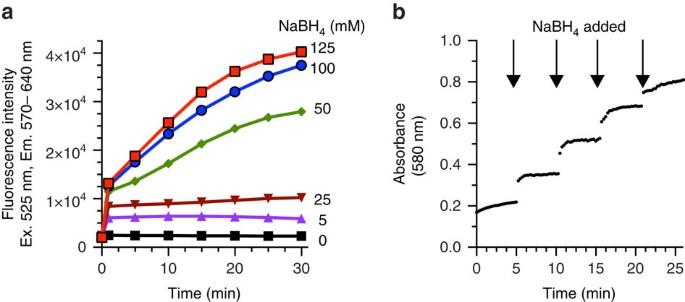Figure 2: Influence of NaBH4on deallylation of RAE. (a) Reaction lifetime dictated by NaBH4concentration. Conditions: 29 μM RAE, 10 p.p.b. Pd(II), 200 μM TFP, 800 mM NH4OAc, 0–125 mM NaBH4, EtOH, 25 °C. (b) Stalled deallylation reaction can be restarted by NaBH4addition. Conditions: 29 μM RAE, 0.3 p.p.m. Pd(II), 200 μM TFP, 800 mM NH4OAc, 0. 0.6, 1.2, 1.8, 2.4 mM NaBH4, added as 2.5 M aliquots at indicated time points. Figure 2: Influence of NaBH 4 on deallylation of RAE. ( a ) Reaction lifetime dictated by NaBH 4 concentration. Conditions: 29 μM RAE, 10 p.p.b. Pd(II), 200 μM TFP, 800 mM NH 4 OAc, 0–125 mM NaBH 4 , EtOH, 25 °C. ( b ) Stalled deallylation reaction can be restarted by NaBH 4 addition. Conditions: 29 μM RAE, 0.3 p.p.m. Pd(II), 200 μM TFP, 800 mM NH 4 OAc, 0. 0.6, 1.2, 1.8, 2.4 mM NaBH 4 , added as 2.5 M aliquots at indicated time points. Full size image Subsequently, we sought to gain insights into the reaction stalling to rationally expand this developing methodology. The Pd-catalysed deallylation of APE stalled in the presence of NH 4 OAc but continued in a phosphate buffer ( Supplementary Fig. 6 ). With 200, 400, 600 and 800 mM NH 4 OAc followed by pH adjustment, the reactions stalled nearly at the same time ( Supplementary Fig. 7 ). The Pd-catalysed deallylation reaction of RAE under a nitrogen atmosphere were found to stall more slowly than those carried out in open air ( Supplementary Fig. 8 ), suggesting that aerobic oxidation of Pd(0) to higher order Pd species may account for the observed reaction stalling. Demonstration of stop-and-go methodology with RAE In an effort to develop a simple, user-friendly colorimetric Pd quantification assay, we prepared a reagent cocktail combining all reaction components except NaBH 4 in a single solution. This cocktail, which is stable for over 2 weeks when stored at 5 °C, can be dispensed as needed, simplifying application of the colorimetric method. The addition of either 20 μl of a solution or 2–5 mg of a solid sample containing trace Pd to 1 ml of the reaction cocktail, followed by the addition of a NaBH 4 solution, generated colour and fluorescence within 1 min. The colour intensity was linearly correlated with Pd concentration, and the dynamic range and reaction time of the assay were tailored by adjusting the NaBH 4 concentration. The power of this method is shown in Fig. 3 . Known concentrations of Pd afford widely different colours with a single concentration of NaBH 4 , with the colour persisting for 24 h ( Fig. 3a ). If a sample contains 1 p.p.b. Pd, then 100 mM NaBH 4 is required to observe a colour change ( Fig. 3b ). If a sample contains 10 p.p.m. Pd, then no NaBH 4 is added to observe a colour change. Thus, Pd concentrations ranging from 1 p.p.b. to 10 p.p.m. (five orders of magnitude) can be distinguished in one reaction solution with NaBH 4 titration. Alternatively, a user may prepare multiple wells with variable NaBH 4 amounts and count a number of coloured wells to estimate the Pd concentrations. 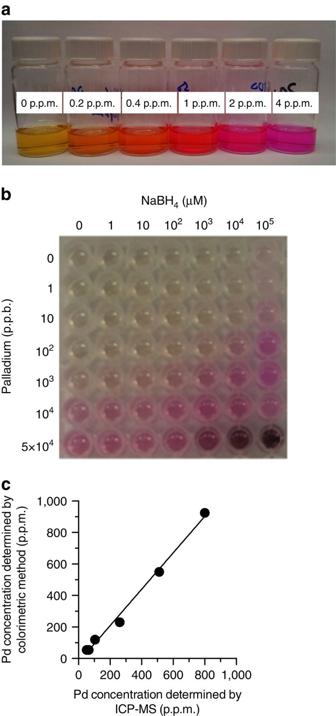Figure 3: Visual quantification of palladium with RAE. (a) The appearance of distinguishable colour correlating to Pd concentration occurs in less than 1 min using a set of Pd standards. Conditions: 29 μM RAE, 0–4.0 p.p.m. Pd, 200 μM TFP, 800 mM NH4OAc, 1.0 mM NaBH4, EtOH, 25 °C. (b) Colorimetric plate showing dependence of colour formation on Pd and NaBH4concentration; 29 μM RAE, 200 μM TFP, 0–50 p.p.m. Pd, 0–100 mM NaBH4, 800 mM NH4OAc 25 °C, EtOH, 10 min,n=3. (c) Conditions: colorimetric analysis as reported inFig. 4a; ICP-MS analysis as reported in the ‘Methods’ section. Figure 3: Visual quantification of palladium with RAE. ( a ) The appearance of distinguishable colour correlating to Pd concentration occurs in less than 1 min using a set of Pd standards. Conditions: 29 μM RAE, 0–4.0 p.p.m. Pd, 200 μM TFP, 800 mM NH 4 OAc, 1.0 mM NaBH 4 , EtOH, 25 °C. ( b ) Colorimetric plate showing dependence of colour formation on Pd and NaBH 4 concentration; 29 μM RAE, 200 μM TFP, 0–50 p.p.m. Pd, 0–100 mM NaBH 4 , 800 mM NH 4 OAc 25 °C, EtOH, 10 min, n =3. ( c ) Conditions: colorimetric analysis as reported in Fig. 4a ; ICP-MS analysis as reported in the ‘Methods’ section. Full size image To confirm that the stop-and-go assay approach is providing quantitative data, we analysed real-world samples. We first tested intermediates used in the preparation of active pharmaceutical ingredients. In pharmaceutical synthesis, reactions may leave behind residual Pd in the products, which is often difficult to remove [13] . Various samples were tested from active projects in the Process and Analytical Chemistry Department at Merck Research Laboratories in which residual Pd removal has proven difficult. Quantification of Pd was initially performed by ICP-MS followed by analysis using RAE. Compared with the ICP-MS analysis, the stop-and-go approach with RAE provided accuracy from 70 to 120%, with residual Pd concentrations ranging from 62 to 800 p.p.m. ( Fig. 3c ). These results were satisfactory for this assay approach to be used for screening dozens of routine Pd remediation protocols. Microscale screening of process adsorbents is often used to identify resins or activated carbons that can be used for selective adsorption of metal impurities in pharmaceutical process research and development [14] [15] . Traditionally, this approach requires close coordination with ICP-MS specialists to allow for quick turnaround time. However, often because of instrument calibration, the vast number of samples, and preparation time, this can be time consuming. As such, the pharmaceutical industry has been interested in a faster technology for trace metal analysis [16] . The application of the colorimetric method enables rapid determination of Pd concentrations ‘on the spot’, in the same laboratory where the process development studies are being carried out. 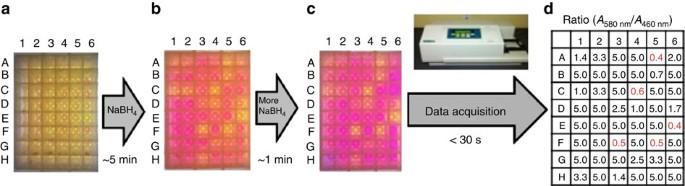Figure 4: Case study of a streamlined process combining adsorbent screening for Pd removal with high-throughput colorimetric Pd detection. (a) Screening kits containing 48 commercial adsorbents15are exposed to a solution of a Pd-containing intermediate. (b) Aliquots from screening kits are evaluated for Pd content using the colorimetric method, as described in protocol. (c) Finding the best potential hits visually by adding more NaBH4. (d) High-throughput mapping of relative Pd concentration by measurement of ultraviolet–visible 570 nm/460 nm using ultraviolet–visible plate reader. Figure 4 shows the results of a high throughput screen of Pd impurity remediation treatments of a pharmaceutical intermediate with 48 metal-scavenging adsorbents, using the stop-and-go assay with RAE to visualize relative Pd levels. An aliquot from each well is treated with the reaction cocktail ( Fig. 4a ), then with NaBH 4 . In less than 5 min, gross differences in Pd concentration are readily apparent to the naked eye by distinguishable colours ( Fig. 4b ). At this point, the reaction had stalled, and too many hits were identified. Accordingly, more NaBH 4 was added to restart the reaction, accentuating the differences between wells and enabling rapid determination of the potential most-effective treatments for residual Pd remediation ( Fig. 4c ). A high-throughput mapping of relative Pd concentration was obtained by plotting the ratio of absorbance at 580 and 460 nm using a ultraviolet–visible plate reader (read time for 48 samples <30 s; Fig. 4d ). These results quantitatively confirm the most effective Pd removal treatments to be wells A5, C4, E6, F3 and F5. Spot-checking several adsorbent treatment samples using conventional ICP-MS showed a good correlation with the colorimetric method, with the selection of the most-effective adsorbent treatments (A5, E6) being identical in both cases. These results demonstrate the utility of a stop-and-go approach in trace metal quantification, providing an important advance for process chemists dealing with remediation of Pd impurity problems using point-of-use high-throughput analysis. Figure 4: Case study of a streamlined process combining adsorbent screening for Pd removal with high-throughput colorimetric Pd detection. ( a ) Screening kits containing 48 commercial adsorbents [15] are exposed to a solution of a Pd-containing intermediate. ( b ) Aliquots from screening kits are evaluated for Pd content using the colorimetric method, as described in protocol. ( c ) Finding the best potential hits visually by adding more NaBH 4 . ( d ) High-throughput mapping of relative Pd concentration by measurement of ultraviolet–visible 570 nm/460 nm using ultraviolet–visible plate reader. Full size image We previously applied APE for quantifying Pd in ore samples without requiring acidic sample digestion [17] , a significant improvement over standard analytical methods such as ICP-MS, but still requiring the use of a blue light source to check fluorescence intensity. This requirement associated with the fluorometric method was not ideal for turbid samples such as ores. Therefore, we applied our colorimetric method for more convenient visualization. We found that the reaction was stalled before effective Pd extraction from the ores, leading to a need to add a large excess of NaBH 4 . However, a 1-min pre-incubation in a DMSO solution of TFP with sonication, followed by the addition of RAE, NH 4 OAc, EtOH and NaBH 4 afforded subpar semi-quantitative data. A second addition of NaBH 4 after the reaction had stalled provided good colorimetric agreement with previous semi-quantitative analysis [17] ( Supplementary Fig. 9 ) within 20 min. Trace Pd is also a significant concern in materials science [18] , [19] . Our colorimetric method could be used to successfully detect trace Pd in polymer materials, as shown in Supplementary Figs 10–12 , Supplementary Table 2 and Supplementary Notes 1 and 2 . Competitive and reversible deactivation in enzymatic assay Horseradish peroxidase (HRP) is a common enzyme for detection and quantification in biological assays [20] , [21] . This enzyme catalytically converts Amplex Red (10-acetyl-3,7-dihydroxyphenoxazine) and H 2 O 2 to resorufin, acetic acid and H 2 O. ( Fig. 5a ) [22] . The reaction continues indefinitely until either Amplex Red or H 2 O 2 is consumed, at which point, signal generation is stopped. 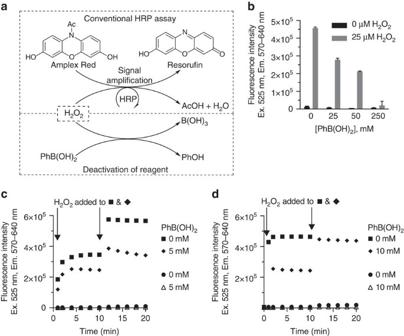Figure 5: Stop-and-go approach in a horseradish peroxidase system. (a) Conversion of Amplex Red to resorufin. (b) Effect of PhB(OH)2on horseradish peroxidase assay. Conditions: 50 μM Amplex Red, 0.1 U ml−1horseradish peroxidase, 25 μM H2O2, 0, 25, 50, 250 mM PhB(OH)2, PBS pH 7.4. (c) Restarting a stopped enzymatic reaction in the presence of an inhibitor. Conditions: 50 μM Amplex Red, 0.05 U ml−1horseradish peroxidase, 0 μM H2O2(0–20 min) for the circle and triangle. For others, 10 μM H2O2at 0 min, 20 μM H2O2at 10 min, PBS pH 7.4. (d) Restarting a stopped enzymatic reaction in the presence of an inhibitor with uninhibited saturation. Conditions: 50 μM Amplex Red, 1 U ml−1horseradish peroxidase, 0 μM H2O2(0–20 min) for the circle and triangle. For others, 10 μM H2O2at 0 min, 30 μM H2O2at 10 min, PBS pH 7.4. After the addition of H2O2at 10 min, the PhB(OH)2-free sample (square) showed a signal above the upper limit of the instrument (above 2 × 106units). Figure 5: Stop-and-go approach in a horseradish peroxidase system. ( a ) Conversion of Amplex Red to resorufin. ( b ) Effect of PhB(OH) 2 on horseradish peroxidase assay. Conditions: 50 μM Amplex Red, 0.1 U ml −1 horseradish peroxidase, 25 μM H 2 O 2 , 0, 25, 50, 250 mM PhB(OH) 2 , PBS pH 7.4. ( c ) Restarting a stopped enzymatic reaction in the presence of an inhibitor. Conditions: 50 μM Amplex Red, 0.05 U ml −1 horseradish peroxidase, 0 μM H 2 O 2 (0–20 min) for the circle and triangle. For others, 10 μM H 2 O 2 at 0 min, 20 μM H 2 O 2 at 10 min, PBS pH 7.4. ( d ) Restarting a stopped enzymatic reaction in the presence of an inhibitor with uninhibited saturation. Conditions: 50 μM Amplex Red, 1 U ml −1 horseradish peroxidase, 0 μM H 2 O 2 (0–20 min) for the circle and triangle. For others, 10 μM H 2 O 2 at 0 min, 30 μM H 2 O 2 at 10 min, PBS pH 7.4. After the addition of H 2 O 2 at 10 min, the PhB(OH) 2 -free sample (square) showed a signal above the upper limit of the instrument (above 2 × 10 6 units). Full size image To illustrate the discontinuous catalysis approach in a different assay, we designed a system in which PhB(OH) 2 would competitively reduce H 2 O 2 ( Fig. 5a ‘Deactivation of reagent’) while the H 2 O 2 -mediated oxidation of Amplex Red occurs (‘Conventional HRP assay’). Figure 5b shows that PhB(OH) 2 was able to do so in a concentration-dependent manner, affording lower signals. Reactions halted by consumption of H 2 O 2 could be restarted by an addition of a fresh aliquot of H 2 O 2 ( Fig. 5c ). With a further addition of H 2 O 2 , signal saturation occurred ( Fig. 5d ). With the inclusion of the competitive scavenger, PhB(OH) 2 to remove H 2 O 2 from the system, the discontinuous catalysis alleviated the problem of overshooting signals, as well as allowed us to restart the reaction without problematic increases in fluorescence ( Fig. 5d ). Although the protocol has not been fully optimized in an HRP system, these data indicate a great potential for the applications of discontinuous catalysis in other enzyme assays. We have developed a competitive and reversible deactivation approach for catalytic quantification assays ( Fig. 6 ). Conversion of RAE to resorufin via a Pd-catalysed Tsuji–Trost reaction is autonomously stalled by the oxidation of reactive Pd(0) to non-reactive species. The addition of NaBH 4 as a reducing agent is able to restart the reaction, enabling accurate measurements over five orders of magnitude. Notably, even in cases where the amount of Pd far exceeds the amount of RAE, the data remain quantitative. We have also demonstrated the utility of the same concept in a widely used HRP assay system, where competitive destruction of H 2 O 2 by PhB(OH) 2 leads to reaction stalling, broadening the dynamic range of the assay. These approaches should be compatible with automation and may find further applicable arenas to broaden the dynamic ranges of catalysis-based assays. 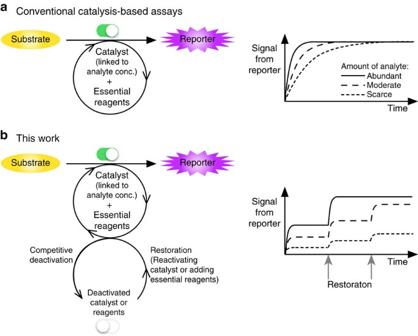Figure 6: Continuous reaction and competitively and reversibly deactivated reaction. (a) Widely used catalytic assays continuously convert a substrate to a reporter molecule. (b) This work presents a stop-and-go paradigm, in which there is a competition between the catalytic reaction and autonomous deactivation of the catalyst (that is, analyte) or the essential reagent. The addition of an activator or a reactant restores the system. Figure 6: Continuous reaction and competitively and reversibly deactivated reaction. ( a ) Widely used catalytic assays continuously convert a substrate to a reporter molecule. ( b ) This work presents a stop-and-go paradigm, in which there is a competition between the catalytic reaction and autonomous deactivation of the catalyst (that is, analyte) or the essential reagent. The addition of an activator or a reactant restores the system. Full size image Ultraviolet–visible spectroscopy The ultraviolet–visible spectra of RAE and resorufin solutions were acquired using a diode array spectrophotometer (Agilent Technologies, Santa Clara, CA) in a quartz cuvette. Other absorbance measurements were recorded in either a 96-well plate using a Modulus II Microplate Multimode reader (Promega, Madison, WI) measuring absorbance at 560 nm or in a clear, round bottom 96-well plates on a Spectra Max M5 spectrometer (Molecular Devices, Sunnyvale, CA) under the control of a Windows-based PC running software pro V5. The samples were analysed at λ =580 nm for the resorufin, and at λ =525 nm for RAE. Fluorescence measurement Fluorescence measurements were read on a Modulus II Microplate Multimode Reader (excitation 525 nm, emission 580–640 nm) or using a HoribaMax Fluorometer (excitation 578 nm, emission 350–700 nm). Metal analysis by ICP-MS The samples were either diluted or suspended directly in concentrated nitric acid or evaporated with a rotary evaporator first and then re-dissolved in concentrated nitric acid for ICP-MS analysis. Depending on the concentration range of the element, either a Perkin-Elmer Elan 6000 quadrupole ICP-MS spectrometer (Perkin-Elmer, Norwalk, CT) or a Thermo Finnigan Element 2 high-resolution ICP-MS spectrometer (Finnigan, Bremen, Germany) was used for the analysis. General protocol for deallylation of RAE A reaction cocktail was prepared by mixing 800 mM NH 4 OAc in EtOH (10 ml) with 800 μM RAE in EtOH (400 μl) and 3 mM TFP in DMSO, with 250 p.p.m. BHT (800 μl). The reaction cocktail (1 ml) was added to individual 2-ml Eppendorf tubes. To half of the samples was added 5% TraceMetal HNO 3 (20 μl) as a control. To the other half of the samples was added a Pd 2+ solution in 5% TraceMetal HNO 3 (20 μl). To all the samples was added NaBH 4 in 10 N NaOH (20 μl). The samples were mixed and transferred (200 μl) to a 96-well black fluorescence well plate. Fluorescence (excitation 525 nm, emission 570–640 nm) was measured every 2 min for 60 min using a Modulus II Microplate Multimode Reader. How to cite this article: Koide, K. et al. A competitive and reversible deactivation approach to catalysis-based quantitative assays. Nat. Commun. 7:10691 doi: 10.1038/ncomms10691 (2016).